Genome-scale metabolic modelling of hepatocytes reveals serine deficiency in patients with non-alcoholic fatty liver disease Several liver disorders result from perturbations in the metabolism of hepatocytes, and their underlying mechanisms can be outlined through the use of genome-scale metabolic models (GEMs). Here we reconstruct a consensus GEM for hepatocytes, which we call iHepatocytes2322 , that extends previous models by including an extensive description of lipid metabolism. We build iHepatocytes2322 using Human Metabolic Reaction 2.0 database and proteomics data in Human Protein Atlas, which experimentally validates the incorporated reactions. The reconstruction process enables improved annotation of the proteomics data using the network centric view of iHepatocytes2322 . We then use iHepatocytes2322 to analyse transcriptomics data obtained from patients with non-alcoholic fatty liver disease. We show that blood concentrations of chondroitin and heparan sulphates are suitable for diagnosing non-alcoholic steatohepatitis and for the staging of non-alcoholic fatty liver disease. Furthermore, we observe serine deficiency in patients with NASH and identify PSPH , SHMT1 and BCAT1 as potential therapeutic targets for the treatment of non-alcoholic steatohepatitis. Hepatocytes have a wide range of physiological functions, including production of bile and hormones, removal of toxic substances, homeostatic regulation of the plasma constituents and synthesis of most plasma proteins [1] . The hepatocytes, the most metabolically active cell types in human, play a major role in overall human metabolism. Deficiency or alterations in the metabolism of hepatocytes can lead to complicated disorders such as hepatitis, non-alcoholic fatty liver disease (NAFLD), cirrhosis and liver cancer, which are serious threats to public health [2] . NAFLD is considered as the hepatic manifestation of obesity and metabolic syndrome, and encompasses a spectrum of pathological changes; ranging from simple fatty liver (FL; steatosis) to non-alcoholic steatohepatitis (NASH) [3] . Even though it is well known that lipid accumulation in the liver is a hallmark of NAFLD [4] , the underlying mechanisms leading to steatosis and further transition to NASH still remain elusive. It is therefore difficult to track the onset and progression or to diagnose and design effective therapeutic techniques. The adverse outcomes of this pathology may possibly be prevented once the molecular mechanisms involved in the metabolism of hepatocytes are deciphered [5] . However, this requires understanding of the coordinated behaviour of a very large number of interconnected metabolic reactions and metabolites. Relating this behaviour with disease and patients have been a major focus in biomedicine [6] . A systems biology approach, based on the employment of genome-scale metabolic models (GEMs), can be used to extend our understanding of these molecular mechanisms, which in turn may enable future therapeutic discoveries [7] , [8] , [9] , [10] . GEMs represent the current knowledge of metabolism generated through the integration of genetic and biochemical studies coupled with cellular, physiological and clinical data [11] . Several generic (non-cell type-specific) GEMs for human metabolism have been previously constructed [12] , [13] , [14] , [15] , [16] . However, neither of these generic networks contain extensive lipid metabolism, which is necessary to study the effect of lipids on the underlying molecular mechanism of NAFLD. Recently, a large-scale GEM for adipocytes, iAdipocytes1809 , with a strong focus on lipid metabolism was presented [17] , and this model can provide a base for further integration of lipid metabolism into generic networks. There is currently no efficient treatment for NASH [18] and new therapeutic approaches are in great demand. This study represents an attempt to rationally identify biomarkers and therapeutic targets using GEM modelling. To reconstruct a high-quality model for hepatocytes, we combine clinical, biochemical and genetic studies such as expression, localization and functional characteristics of the proteins. We first significantly expand the content of our Human Metabolic Reaction (HMR) database by including extensive lipid metabolism and generate HMR 2.0 database. This represents an important step forward, as lipids have major effect on the development of NAFLD and other metabolic diseases [19] . Second, we reconstruct a consensus GEM for hepatocytes, iHepatocytes2322 , by using the HMR 2.0 database and large-scale proteomics data. We also merge previously published hepatocyte models to cover the entire known metabolic functions of hepatocytes and incorporated additional clinical data (for example, liver tissue and plasma fatty acid (FA) contents in lipid structures). During the reconstruction process, we reevaluate the hepatocyte proteomics data after identifying proteins that are included in the model to ensure network connectivity, but are assessed as absent in hepatocytes in the Human Protein Atlas (HPA, http://www.proteinatlas.org ) [20] . Finally, we employ iHepatocytes2322 for the analysis of differential gene expression data from liver tissues of subject groups with NAFLD. This lead to new insights into the molecular mechanisms involved in NASH, which are used for the identification of potential metabolic biomarkers and therapeutic targets for treatment of NASH ( Fig. 1 ). 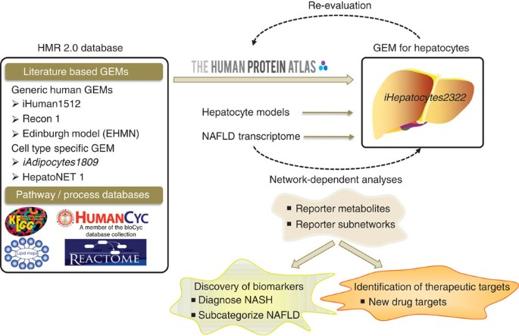Figure 1: Effective therapeutic approach through GEM modelling. Schematic illustration of how a consensus GEM for hepatocytes,iHepatocytes2322, may contribute to the development of effective therapeutic approaches for NAFLD patients. The HMR 2.0 database was constructed through the use of previously published GEMs and pathway databases, including KEGG, HumanCyc, Reactome and LIPIDMAPS Lipidomics Gateway. Elements of lipid metabolism were included in the HMR database to understand the effect of the lipids and their interactions during the appearance of NAFLD. The HMR 2.0 database was used for reconstruction ofiHepatocytes2322based on proteomics data in the HPA, transcriptomics data in NAFLD patients and previously published hepatocytes models. During the reconstruction process,iHepatocytes2322was employed for the improvement of proteomics data through identification and re-annotation of putative false-negative proteins. The resulting GEM was used for the analysis of clinical data obtained from NAFLD patients to investigate the alterations in their hepatocyte metabolism and eventually for the discovery of biomarkers and identifying therapeutic targets. Through our systems biology-based analysis, potential biomarkers for diagnosing NASH and for subcatogorizing NAFLD patients were discovered. Furthermore, a list of candidate therapeutic targets was identified to develop efficient treatments for NASH patients. Figure 1: Effective therapeutic approach through GEM modelling. Schematic illustration of how a consensus GEM for hepatocytes, iHepatocytes2322 , may contribute to the development of effective therapeutic approaches for NAFLD patients. The HMR 2.0 database was constructed through the use of previously published GEMs and pathway databases, including KEGG, HumanCyc, Reactome and LIPIDMAPS Lipidomics Gateway. Elements of lipid metabolism were included in the HMR database to understand the effect of the lipids and their interactions during the appearance of NAFLD. The HMR 2.0 database was used for reconstruction of iHepatocytes2322 based on proteomics data in the HPA, transcriptomics data in NAFLD patients and previously published hepatocytes models. During the reconstruction process, iHepatocytes2322 was employed for the improvement of proteomics data through identification and re-annotation of putative false-negative proteins. The resulting GEM was used for the analysis of clinical data obtained from NAFLD patients to investigate the alterations in their hepatocyte metabolism and eventually for the discovery of biomarkers and identifying therapeutic targets. Through our systems biology-based analysis, potential biomarkers for diagnosing NASH and for subcatogorizing NAFLD patients were discovered. Furthermore, a list of candidate therapeutic targets was identified to develop efficient treatments for NASH patients. Full size image HMR 2.0 database To provide a resource for automated and semi-automated reconstruction of cell-type-specific GEMs, we previously constructed the HMR database [15] . This comprehensive database, together with the INIT (Integrative Network Inference for Tissues) algorithm, have been employed for automated generation of cell-type-specific GEMs [15] . These models form the basis for the Human Metabolic Atlas ( http://www.metabolicatlas.org ), which is a web-based resource for human metabolism. Here we expanded the HMR database by incorporating extensive lipid metabolism, which accounts for individual FAs rather than relying on generic FAs pool metabolite. The generated HMR 2.0 database is formulated using 59 FAs ( Supplementary Table 1 ), which enables mapping and integration of lipidomics data. Integration of extensive lipid metabolism (for example, formation of lipid droplets (LDs) and lipoproteins) may allow not only for understanding the contribution of lipids to the development of diseases but also allow for study of the relationship between lipid metabolism and cellular molecular mechanisms [17] . 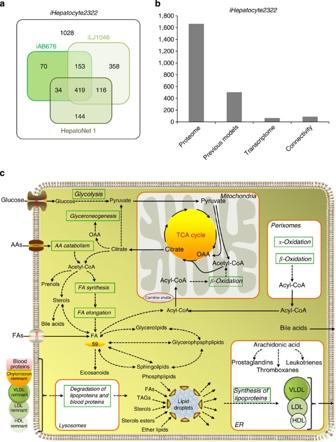Figure 2: Consensus GEM for hepatocytes,iHepatocytes2322. (a)iHepatocytes2322is reconstructed through the use of the HMR 2.0 database and improved annotation of proteomics data in the HPA. This high-quality model includes the structure of major lipid metabolism in hepatocytes, as well as all of the reactions and associated genes to those reactions in previously published GEM for hepatocytes. The overlapping of the genes iniHepatocytes2322and previously published models are presented. One thousand and twenty-eight new protein-coding genes were included intoiHepatocytes2322primarily based on proteomics evidence provided by HPA. (b) Genes and associated reactions iniHepatocytes2322are included into the model based on the high-quality proteome, transcriptome, previously published models, as well as the connectivity. The overall distribution is shown. (c)iHepatocytes2322contains extensive lipid metabolism that is known to exist in hepatocytes, in addition to other known metabolic pathways. In the model, 59 different individual FAs are used to allow the integration of high-quality lipidomics data rather than generic pool names. The model can uptake the remnants of chylomicrons, VLDL, low-density lipoproteins (LDLs) and high-density lipoproteins (HDLs) and can form and degrade LDs. Moreover, the model can synthesis VLDL, LDL and HDL, and secrete it to the blood. Some of the important elements of lipid metabolism are shown. Reactions are included in the HMR 2.0 database depending on evidence from previously published models and databases ( Supplementary Table 2 ) or on the availability of specific experimental evidence for the occurrence of the reaction. The reaction–gene associations of the generic human network were improved based on the publically available resources and literature review. The HMR 2.0 database is the largest biochemical reaction database for human metabolism in terms of number of reactions/genes/metabolites, as well as in terms of covering most parts of metabolism. Consensus GEM for hepatocytes and improved proteome annotation Cell-type-specific GEMs can be employed for the analysis of high-throughput patient (-omics) data, simulation of the metabolic differences under health and disease states, and eventually for predicting the cellular phenotype [10] . Previously, several GEMs for hepatocytes, including HepatoNET 1 (ref. 1 ), iLJ1046 (ref. 21 ), iAB676 (ref. 22 ) and iHepatocyte1154 (ref. 15 ) have been reconstructed. Here we generated a consensus GEM for hepatocytes, iHepatocytes2322 , based on proteomics data ( Supplementary Data 1 ) and the updated HMR 2.0 database. iHepatocytes2322 contains all of the protein-coding genes and associated reactions in previously published liver models ( Fig. 2a ). In addition to the proteomics data and previous models, protein-coding genes are also included in iHepatocytes2322 based on transcriptomics data and connectivity ( Fig. 2b ). Reactions and associated proteins were assigned into eight different compartments following our HMR database standard based on the subcellular localization of the proteins in HPA and Uniprot. The protein localization information in HPA and Uniprot were assigned to relevant compartments in the HMR 2.0 database ( Supplementary Data 2 ). A confidence score for each protein was calculated based on the availability of knowledge in HPA and Uniprot ( Supplementary Data 3 ). Furthermore, the connectivity in the model was checked carefully, such that all metabolites consumed in one reaction should be able to be produced by another reaction or they should be taken up from the plasma. Finally, additional clinical data for plasma and hepatocyte lipid concentrations for individual FAs were incorporated into the model ( Supplementary Data 4 ). Figure 2: Consensus GEM for hepatocytes, iHepatocytes2322 . ( a ) iHepatocytes2322 is reconstructed through the use of the HMR 2.0 database and improved annotation of proteomics data in the HPA. This high-quality model includes the structure of major lipid metabolism in hepatocytes, as well as all of the reactions and associated genes to those reactions in previously published GEM for hepatocytes. The overlapping of the genes in iHepatocytes2322 and previously published models are presented. One thousand and twenty-eight new protein-coding genes were included into iHepatocytes2322 primarily based on proteomics evidence provided by HPA. ( b ) Genes and associated reactions in iHepatocytes2322 are included into the model based on the high-quality proteome, transcriptome, previously published models, as well as the connectivity. The overall distribution is shown. ( c ) iHepatocytes2322 contains extensive lipid metabolism that is known to exist in hepatocytes, in addition to other known metabolic pathways. In the model, 59 different individual FAs are used to allow the integration of high-quality lipidomics data rather than generic pool names. The model can uptake the remnants of chylomicrons, VLDL, low-density lipoproteins (LDLs) and high-density lipoproteins (HDLs) and can form and degrade LDs. Moreover, the model can synthesis VLDL, LDL and HDL, and secrete it to the blood. Some of the important elements of lipid metabolism are shown. Full size image iHepatocytes2322 differs from previously published hepatocyte GEMs primarily in terms of coverage in lipid metabolism. Among the new lipid-related functions are uptake of the remnants of lipoproteins (chylomicrons, very-low-density lipoprotein (VLDL),low-density lipoproteins and high-density lipoproteins), the formation and degradation of LDs and secretion of synthesized lipoproteins (VLDL, low-density lipoprotein and high-density lipoprotein; Fig. 2c ). We tested iHepatocytes2322 by simulating 256 different biologically defined metabolic functions (for example, the synthesis of FAs, amino acids, cholesterol and bile acids; Supplementary Data 5 ) that is known to occur in hepatocytes using the RAVEN Toolbox [23] . Furthermore, the ability of iHepatocytes2322 for performing gluconeogenesis was demonstrated using experimentally measured secretion rates for glucose and albumin, and uptake rates for glycerol, lactate, amino acids and FAs in primary rat hepatocytes [24] ( Supplementary Data 6 ). The HPA covers the annotated expression of proteins and their subcellular localization in major human cell types, cancer and cell lines [20] . Relative abundance of proteins encoded by 15,155 genes in hepatocytes was analysed with 18,707 high-throughput-generated affinity-purified antibodies ( Supplementary Data 1 ). The model reconstruction process was in excellent agreement with the protein profiling of hepatocytes in HPA. During the implementation of the metabolic tasks in iHepatocytes2322 , merely 61 (~1,6%) out of 3,765 proteins in the HMR database and associated reactions had to be integrated into the model to maintain the functionality, even though they have been reported to be non-expressed in hepatocytes according to the HPA. We re-analysed the immunohistochemistry (IHC) data of these 61 proteins and found that 20 (0.5%) of these proteins actually should display presence in the liver ( Supplementary Data 7 ). Initial disconcordant data were due to the suboptimal titration of the antibody, misinterpretation of weak IHC staining or due to interference with other cell types besides hepatocytes present in the liver (for example, Kupffer cells and sinusoids). Nine (0.2%) of the investigated proteins showed more concordant results to the mathematic model when re-analysed using another antibody targeting the same protein. Fifteen proteins (0.4%) with negative IHC data were kept as negative in HPA data, as limited literature was available and/or concordant results were seen in subsets of the remaining panel of tissues included in the HPA high-throughput setup. The remaining 17 proteins (0,5%) were inaccurately assessed by IHC due to technical issues, such as antigen recognition due to antigen conformational changes, fixation or suboptimal antibody. Discovery of biomarkers for NASH NAFLD is progressively diagnosed worldwide [25] , is tightly associated with obesity, type 2 diabetes, insulin-resistance and hypertension, and represents a severe risk for the development of cirrhosis and hepatocellular carcinoma [26] . Despite its severe drawbacks, liver biopsy is still the most common procedure for diagnosing NASH [18] . Thus, there is a need for identifying non-invasive biomarkers to diagnose NASH and to subcategorize the NAFLD patients without taking biopsies. To date, there has been a number of studies aiming at finding non-invasive biomarkers for diagnosis and staging of NAFLD [27] , [28] . A routinely available biochemical marker for hepatocellular damage is alanine transferase, but this has only proven to have moderate diagnostic value. Other markers for metabolic syndrome (such as adiponectin or leptin), inflammation (such as tumour-necrosis factor-α or interleukin 6), oxidative stress (such as catalase, glutathione peroxidase and overall plasma ferric reducing ability), apoptosis and fibrosis have also been proposed as biomarkers for staging NAFLD [29] , [30] . Among these, the apoptosis markers are arguably the ones with the best predictive ability. One such marker is cytokeratin 18 fragment, which is an intermediate filament expressed in single-layer epithelial tissues in patients with NAFLD. Its strong correlation with the occurrence of liver fibrosis and hepatic inflammation has been reported [31] , [32] . In this study, we focused on predicting potential metabolite biomarkers rather than on proteins, as they can quickly and easily be measured both in the plasma and urine [33] . We analysed the liver gene expression data obtained from NASH (severe stage of NAFLD) patients ( Supplementary Fig. 1 ) to understand the multi-factorial nature of its appearance by using iHepatocytes2322 as a scaffold for data analysis. The liver transcriptomics data include samples from 45 different subjects, and the samples were diagnosed as healthy ( n =19), steatotic ( n =10), NASH with FL ( n =9) and NASH without FL ( n =7) [34] . Diagnosis of the liver samples was first established by a Liver Tissue Cell Distribution System medical pathologist and was confirmed by histological examination at the University of Arizona in a blinded fashion. Steatosis was diagnosed by >10% fat deposition without inflammation or fibrosis. NASH with and without FL samples were characterized by >5% fat deposition and <5% fat deposition within hepatocytes, respectively, and both were accompanied by inflammation and fibrosis. The severity can be ordered as NASH without FL>NASH with FL>steatotic>healthy. Clinical information of these human liver samples has been described previously [35] . In brief, samples of frozen and formalin-fixed, paraffin embedded adult explant livers were obtained from the Liver Tissue Cell Distribution System at the University of Minnesota, Virginia Commonwealth University, and the University of Pennsylvania. Histological staining of progressive stages of NAFLD were provided for each human liver donor samples using a previously established scoring system [36] , and representative images of haematoxylin and eosin-stained livers from normal, steatotic, NASH with FL and NASH without FL have been provided [35] . The age, gender and disease state of the patients are included in Supplementary Data 8 . We identified metabolic differences by performing a pair-wise analysis of the gene expression of subjects with NASH with and without FL versus healthy ( Fig. 3 ) and steatotic ( Supplementary Fig. 2 ) samples using the Reporter Metabolite algorithm [37] . Reporter Metabolite analysis allows for the identification of metabolites in the network for which there is significant enrichment of associated gene expression changes. Such metabolites can therefore be used to discover key regions of the metabolic network, which are significantly perturbed between the compared conditions [37] . The analyses for two NASH patient groups were performed independently and a total of 60 statistically significant (Reporter Features, P -value <0.05) Reporter Metabolites for NASH with and without FL versus healthy samples were identified. The association of the Reporter Metabolites with up- and downregulated genes and their metabolic subsystems classified in the HMR database are presented ( Fig. 3 ). NASH is associated with some well-studied major metabolic abnormalities. These include increased uptake of FAs, decreased β-oxidation and cholesterol synthesis, and irregular preparation and export of triacylglycerols and cholesterol in the form of VLDL particles [38] , [39] . Many of the metabolites associated with these functions were identified in our analysis, and literature evidence for their association with the appearance of NAFLD are included in Supplementary Data 9 . 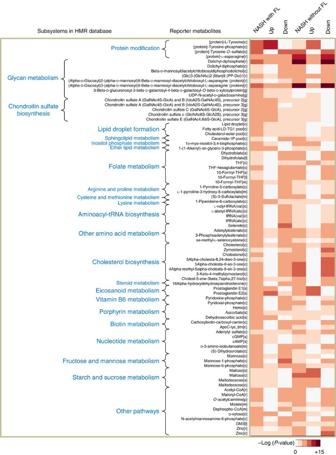Figure 3: Reporter Metabolites through the global analysis of high-throughput data. Metabolic differences between the liver gene expression profiles of subjects with NASH with and without FL, and healthy subjects were investigated through the employment ofiHepatocytes2322.In addition to the reporter metabolites associated with the known pathways involved in the appearance of NASH, reporter metabolites associated with the less well-studied subsystems, including Glycan metabolism and CS metabolism have been discovered. The blood level of CS, which can be secreted and taken up by the blood, is identified as a candidate biomarker for diagnosing NASH and staging NAFLD.P-values for each reporter metabolite were calculated for up- and downregulated genes, and minus logarithm of theP-values are presented. Figure 3: Reporter Metabolites through the global analysis of high-throughput data. Metabolic differences between the liver gene expression profiles of subjects with NASH with and without FL, and healthy subjects were investigated through the employment of iHepatocytes2322. In addition to the reporter metabolites associated with the known pathways involved in the appearance of NASH, reporter metabolites associated with the less well-studied subsystems, including Glycan metabolism and CS metabolism have been discovered. The blood level of CS, which can be secreted and taken up by the blood, is identified as a candidate biomarker for diagnosing NASH and staging NAFLD. P -values for each reporter metabolite were calculated for up- and downregulated genes, and minus logarithm of the P -values are presented. Full size image We focused here on the less well-studied metabolic subsystems involved in the progression of the NASH. In addition to subsystems previously implicated in NASH (for example, folate, vitamin B6, lipid, eicosanoid and amino acid metabolism [40] , [41] ), new Reporter Metabolites involved in glycan metabolism and biosynthesis of chondroitin sulphate (CS), a proteoglycan (PG) were identified. Previously, the association of serum levels of hyaluronic acid (a non-sulphated glycosaminoglycan) with the fibrosis stage in chronic liver diseases, including NAFLD, was reported [28] , [42] . Hyaluronic acid is distributed throughout epithelial tissues and most of its disassembly takes place in endothelial liver cells. Fibrosis and cirrhosis lead to impaired clearance of hyaluronic fragments due to the lack of function in endothelial liver cells. Kalsch et al . [43] re-evaluated the hyaluronic acid as biomarkers for NAFLD and fibrosis in a cohort of 127 patients, and compared these results with the histological diagnosis of NAFLD. PGs are composed of glycosaminoglycans, including CS and heparan sulphate (HS) and core proteins. The biosynthesis of PGs starts with the xylosylation of serine residues in core proteins. To gain more knowledge about the metabolic differences around PGs, the detailed CS and HS biosynthesis pathway and the gene expression changes in NASH with and without FL patients versus healthy subjects are presented ( Supplementary Fig. 3 ). It is observed that the expression of the genes involved in the CS biosynthesis are upregulated, whereas the expression of genes involved in the biosynthesis of HS are downregulated ( Supplementary Table 3 ). It has been earlier reported that CSPG2 gene is upregulated in biopsy-proven NASH patients versus obese controls [44] . CS and HS were also implicated in cancer progression [45] , one of the most severe outcomes of NASH. Therefore, we predicted that these changes in gene expression, in particular as it involves complete metabolic pathways, may correlate with a change in blood concentration of the pathway-associated metabolites. Hence, the blood level of CS and HS can be regarded as a potential biomarker for diagnosing NASH. To validate the gene expression changes around CS and HS, we retrieved another microarray data set that includes liver samples from eight patients with morbid obesity and associated NASH, and seven control obese subjects from the Gene Expression Omnibus public repository under the accession number GSE37031 . The control subjects had normal serum aminotransferase levels and liver histology. The Reporter Metabolites for this data set are presented ( Supplementary Fig. 4 ). As can be seen, there are quite large differences in terms of overlap with the previously used data set. This can most likely be attributed to the small sample sizes in both data sets. Most importantly though, CS were found among the top-ranking metabolites for which there were transcriptional upregulation, and HS were found among the top-ranking metabolites for which there were transcriptional downregulation (Reporter Features, P -value <0.05). Potential therapeutic targets for NASH The Reporter Subnetwork algorithm identifies a set of metabolic reactions that exhibit transcriptional correlation after a perturbation (in this case NASH) [37] . We applied this algorithm to gain more insights into the molecular mechanisms involved in the appearance of NASH. 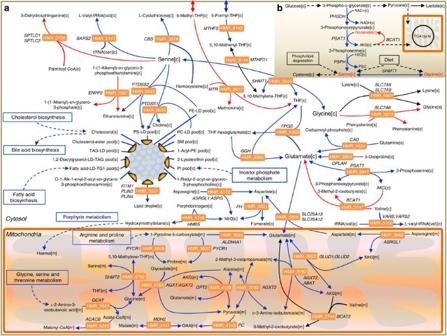Figure 4: Reporter Subnetworks through mapping of high-throughput data. (a) Reporter Subnetworks were identified iniHepatocytes2322through the pair-wise comparison of liver transcriptomics data obtained from NASH with and without FL versus healthy subjects. Amino acids, in particular serine, glutamate and glycine, have a role in the appearance of NASH, and the significant changes around these amino acids have been presented. Through our analysis, three different drug targets (PSPH,SHMT1andBCAT1) have been identified. Red arrows indicate overexpression of the associated genes, whereas blue arrows indicate underexpression. PS is presented as PS–LD pool in the subnetwork and the descriptions for other metabolites are included in the SBML (Systems Biology Mark-up Language) model file. (b) Serine is endogenously biosynthesized from 3-phospho-D-glycerate and glycine. It can also be derived from the diet and the degradation of protein and/or phospholipids. After removing highly connected metabolites (for example, cofactors; Supplementary Table 4 ) in iHepatocytes2322 , the involved subnetworks in either NASH with or without FL were identified and they are presented ( Fig. 4a and Supplementary Fig. 5 ). The enzymes involved in the reactions are also represented ( Fig. 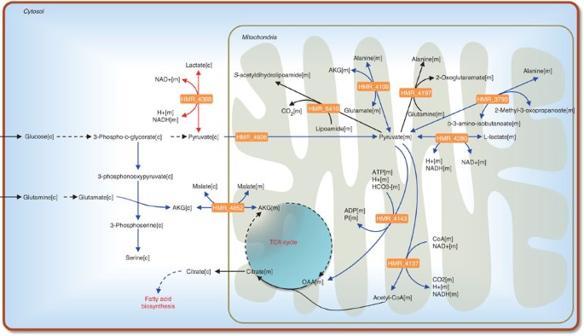Figure 5: Mitochondrial dysfunction in NASH. Mitochondrial reactions involving pyruvate as a reactant iniHepatocytes2322are presented. Arrows are coloured based on the direction of change in expression of the corresponding genes in NASH with and without FL samples versus healthy samples. Red arrows indicate overexpression of the associated genes, whereas blue arrows indicate underexpression. Not statistically significant changes (t-test,P-value >0.05) associated to the reactions are indicated with black arrows. 4a ), and related P -values and fold changes of their expression are shown ( Supplementary Table 5 ). Figure 4: Reporter Subnetworks through mapping of high-throughput data. ( a ) Reporter Subnetworks were identified in iHepatocytes2322 through the pair-wise comparison of liver transcriptomics data obtained from NASH with and without FL versus healthy subjects. Amino acids, in particular serine, glutamate and glycine, have a role in the appearance of NASH, and the significant changes around these amino acids have been presented. Through our analysis, three different drug targets ( PSPH , SHMT1 and BCAT1 ) have been identified. Red arrows indicate overexpression of the associated genes, whereas blue arrows indicate underexpression. PS is presented as PS–LD pool in the subnetwork and the descriptions for other metabolites are included in the SBML (Systems Biology Mark-up Language) model file. ( b ) Serine is endogenously biosynthesized from 3-phospho- D -glycerate and glycine. It can also be derived from the diet and the degradation of protein and/or phospholipids. Full size image The Reporter Subnetwork analysis showed that the non-essential amino acids serine, glycine, glutamate, glutamine, aspartate, asparagine and alanine, and the essential amino acid valine and methionine seem to be involved in the appearance of NASH. For reasons discussed later, serine, glycine and glutamate are of particular interest. Several metabolites involved in folate metabolism (for example, tetrahydrofolate (THF), 5-methyl-THF, 5-formyl-THF, 5,10-methenyl-THF and 5,10-methylene-THF) were also identified in the Reporter Subnetwork analysis, and these metabolites are involved in the interconversion of serine, glycine and glutamate. The metabolism around THF changed in NASH patients and this difference may be dependent on the uptake of 5-methyl-THF and 5-formyl-THF. Moreover, phosphatidylserine (PS), an essential component for formation of LDs, was identified through our analysis. LDs have diverse roles in the cell, such as serving as storage for triacylglycerols and CEs, or protecting the cell from excess lipids or lipophilic substances that may be toxic [46] . The enzymes PS synthases PTDSS1 and PTDSS2 that catalyse the production of PS by condensation of phosphatidylcholine and phosphatidylethanolamine, respectively, were significantly downregulated in NASH patients. The significant changes in the level of PS in cirrhotic (severe stage of NASH) livers was previously reported in a study on changes in lipid species in subjects with cirrhotic livers compared with healthy controls [47] . Given that PS is essential for hepatocytes, we hypothesize that decreased activity of these enzymes may be associated with a decrease in the endogenous level of serine, which is the second most connected node in our identified Reporter Subnetworks ( Fig. 4a ). Serine is endogenously biosynthesized from a glycolytic intermediate, 3-phospho- D -glycerate. This three-step process is catalysed by phosphoglycerate dehydrogenase ( PHGDH ), phosphoserine aminotransferase 1 ( PSAT1 ) and phosphoserine phosphatase ( PSPH ), as shown in Fig. 4b . An alternative synthesis pathway is via the reversible interconversion with glycine through hydroxymethyltransferases SHMT1 and SHMT2 . Serine can also be derived from the diet and the degradation of protein and/or phospholipids. Serine plays a key role in the central metabolism, where it is involved in the formation of macromolecules, including lipids (sphingosine and PS), and other building blocks and cofactors, such as protein (glycine and cysteine), creatine, porphyrins, glutathione and nucleotides [48] . Through differential analysis of transcriptomics data from the NASH patients, it was also observed that gene expression of several enzymes that either use serine as substrate or produce it as a product, including CBS (cysteine synthesis), SARS2 (aminoacyl-tRNA biosynthesis), SHMT1 and SHMT2 (glycine synthesis) were significantly downregulated ( t -test, P -value <0.05), whereas SPTLC1 and SPTLC2 (sphingosine synthesis) were significantly upregulated ( Supplementary Table 5 ). Downregulation of CBS that catalyses the conversion of serine and homocysteine to L -cystathionine and upregulation of MTR that condensates homocysteine to methionine through the use of 5-methyl-THF indicate that there are metabolic changes around homocysteine in NASH patients. Notably, it has been earlier reported that the plasma homocysteine level can be used for diagnosing NASH and classifying steatosis and NASH patients [49] . It is not always straightforward to relate blood concentrations to gene expression levels of the involved enzymes, but our model-based analysis suggests a mechanistic explanation for this. Taken together, the results suggest that the changes in the level of PS in the liver [47] as well as the relative increase in the homocysteine blood level [49] is caused by decreased level of endogenous serine. To test this hypothesis, we checked the expression level of enzymes that catalyse the biosynthesis of serine in the liver of NASH patients, and it was observed that the expression levels of PHGDH , PSAT1 , PSPH in serine synthesis pathway (SSP), and SHMT1 and SHMT2 enzymes were significantly downregulated ( Supplementary Table 6 ). Decreased levels of serine in NASH patients was supported by plasma profiling of amino acids, where the serine level in the plasma is relatively decreased (15% decrease, P -value=0.0568) compared with healthy subjects [50] . Equimolar amounts of serine and alpha-ketoglutarate (AKG) are synthesized in the SSP, and downregulation of reactions in SSP decrease the anaplerosis of AKG to the tricarboxylic acid (TCA) cycle in the form of glutamate [51] . Decreased level of serine also causes an accumulation of upstream glycolytic intermediates [52] , and a decreased flux of mitochondrial AKG is compensated by an increased flux of pyruvate to oxaloacetate in a healthy cell. To investigate the occurrence of this mechanism in NASH patients, we examined all mitochondrial reactions involving pyruvate as reactant in iHepatocytes2322 . We found that the corresponding genes were downregulated for five out of seven such reactions ( Fig. 5 and Supplementary Table 7 ). Furthermore, we investigated the expression of level of mitochondrial pyruvate carriers ( MPC1 and MPC2 ) and mitochondrial AKG/malate carrier ( SLC25A11 ), and it was observed that their expression levels were downregulated in NASH patients. These indicate that the mitochondrial metabolic activity (TCA cycle) of hepatocytes is decreased in NASH patients in comparison with healthy subjects. This is in agreement with findings in our previous study wherein we investigated the metabolic changes in the case of fat accumulation in adipocytes in response to obesity [17] . Figure 5: Mitochondrial dysfunction in NASH. Mitochondrial reactions involving pyruvate as a reactant in iHepatocytes2322 are presented. Arrows are coloured based on the direction of change in expression of the corresponding genes in NASH with and without FL samples versus healthy samples. Red arrows indicate overexpression of the associated genes, whereas blue arrows indicate underexpression. Not statistically significant changes ( t -test, P -value >0.05) associated to the reactions are indicated with black arrows. Full size image In the appearance of NASH, glutamate, which is the most connected node in our Reporter Subnetwork, plays a significant role as well. All enzymes linked to glutamate, except the branched chain amino-acid transaminase 1 ( BCAT1 ) that convert AKG and valine to glutamate in the cytosol, are downregulated. In NASH patients, upregulation of BCAT1 is previously reported [40] and our study identifies its mechanism in the appearance of NASH. The simultaneous upregulation of BCAT1 and downregulation of PSPH could point to an imbalance in intercellular level of AKG and glutamate. This could possibly result in an accumulation of intracellular glutamate, which would then be compensated for by reduced uptake from/increased export to the blood. Notably, a previous study detected a significantly higher level of glutamate (60% increase, P =9.808E−09) in the plasma profiling of the amino acids in NASH patients [50] . At the same time, this may result in a higher demand for valine in hepatocytes, and given that valine is an essential amino acid this would arguably correlate with an increased uptake. Indeed, the same study [50] reported that the plasma valine concentration displayed significant changes (10% increase, P -value=0.012). To gain insights into the underlying molecular mechanisms of NASH, we reconstructed a consensus GEM for hepatocytes, which allowed for study of the interactions between lipid metabolism and other cellular metabolic functions. The reconstruction process enabled re-evaluation and improved annotation of the proteomics data, and our analysis clearly showed the power of using reconstructed metabolic networks for improving the annotation of experimental expression data. This highly curated GEM reconstructed through the use of the HMR 2.0 database enables interpretation of systemic effects, provides deeper insight into omics data for better understanding of the genotype–phenotype relationship in NASH subjects and allows for application of constraint-based modelling techniques to distinguish the NASH-specific metabolic features. On the basis of liver transcriptomics data of NASH patients and systems biology-based approaches, we proposed potential biomarkers and identified candidate therapeutic targets for NASH. Throughout our analysis, the gene expression levels served only as cues for the changes in the metabolic flux of its associated reaction. It is known that the correlation between these measurements is known to be limited, but several methods for inferring flux rates using gene expression data have been successfully applied [53] , [54] . On the basis of our analysis, increasing the serine level in hepatocytes through the uptake of serine as a dietary supplement could be beneficial for NASH patients. Similarly, activity loss of PHGDH in SSP in the brain, which causes low serine and glycine levels, and affects neuronal function, is reversed by serine supplementation [55] . The toxicity and the dosage of serine during its uptake through diet have been previously studied. Furthermore, long-term serine treatment decreased the homocysteine level in animal studies [56] and in humans, in a single-dose situation [57] . One other possible way to increase the serine level to offer the possibility for therapeutic interventions is activation of the enzymes in SSP or SHMT1 and SHMT2 that converts glycine to serine. Three different enzymes constitute the SSP and it is earlier reported that PSPH is the rate-controlling enzyme for SSP in the liver [58] . Activation of the SSP through the amplification of PSPH may also decrease the flux through pyruvate and lactate formation in cytosol, as increased pyruvate and lactate levels were previously reported in NASH patients [50] . Recently, Frayling et al . [59] performed a genome-wide association study using 1,004 non-diabetic individuals and identified 8 common genetic variants relevant to insulin sensitivity and type 2 diabetes that are strongly linked to NASH phenotype. Their findings are in agreement with our results and they reported that three variants were associated with serine levels, out of which one is in the PHGDH gene and the other two are independently in the PSPH gene. Boosting the serine level through SSP will also increase the flux on unregulated anaplerotic reactions that drive glutamine-derived carbon (via glutamate) into the TCA cycle through increased level of AKG and result in increased TCA cycle flux [51] . TCA cycle intermediates, besides being involved in driving energy production, are also used for biosynthesis of lipids (citrate), porphyrin (succinyl-CoA) and amino acids (AKG and oxaloacetate). AKG concentration in the cytosol can also be increased by inhibition of BCAT1 , which converts AKG and valine to glutamate. Increasing the AKG level by either overexpressing PSPH or inhibiting BCAT1 may change the NASH-specific patterns to healthy patterns, and it may potentially be used to develop an effective treatment for NASH. In conclusion, we reconstructed a consensus GEM for hepatocytes, showed how reconstructed metabolic networks can be used for improving the annotation of experimental data and employed the model to gain more insight into the metabolic transformations associated with the development of NASH. Our analysis suggests that it is possible to diagnose NASH through identified metabolic biomarkers such as CS and HS levels in the blood. Furthermore, the development of therapeutic techniques based on the enhancement of endogenous serine and AKG levels may correct the underlying aetiology of NASH. This could be achieved by activation (or elevated expression) of PSPH and SHMT1 , and inhibition of BCAT1 . This study demonstrates that a deeper understanding of the metabolic changes obtained through GEM modelling may allow for elucidating the unknown aetiology of NASH, discovery of novel biomarkers, identification of drug targets and, eventually, development of efficient treatment strategies. Expansion of HMR database The HMR database was constructed [15] by integrating the elements of stoichiometric networks of human metabolism, Recon 1 (ref. 12 ) and EHMN [13] , [14] , as well as the Kyoto Encyclopedia of Genes and Genomes (KEGG) database [60] . To generate a generic network for studying the effect of the lipids on the cellular metabolism, we expanded the coverage of the HMR database. We first merged metabolism of lipids and lipoproteins in Reactome, a manually curated and peer-reviewed pathway database [61] , and the literature-based GEMs including Recon 1 (ref. 12 ), EHMN [13] , [14] and HepatoNet 1, a manually reconstructed GEM for hepatocytes [1] . Extensive lipid metabolism involving 59 different FAs in the comprehensive database for lipid biology for mammalian cells, Lipidomics Gateway [62] , were included in the network and the gaps in the resulting network were filled using public databases such as KEGG [60] and HumanCyc [63] . The resulting generic human GEM is called HMR 2.0 database, and to ensure the standardization of the HMR database all model components were extensively annotated with database identifiers. HMDB, Lipid Map [62] , KEGG and ChEBI identifiers were assigned for each metabolite, and KEGG ids and enzyme commission numbers were assigned for each reaction. Alternative genes associated to reactions were assigned using UniProt [64] and Lipid Map proteome database [65] using enzyme commission numbers. The resulting HMR database contains 3,765 genes, 6,007 metabolites (3,160 unique metabolites) and 8,181 reactions, and 74% of the reactions associated to one or more genes. The generated HMR 2.0 database is the most comprehensive resource for the human-related biochemical reactions and includes all of the genes, metabolites and reactions in the recently published models ( Supplementary Table 8 ). It also includes all of the genes and associated reactions in recently published generic human model Recon2 (ref. 16 ). In the HMR 2.0 database, proteins encoded by genes are classified into eight different compartments, including cytosol, nucleus, endoplasmic reticulum, Golgi apparatus, peroxisome, lysosome, mitochondria and extracellular space. The HMR 2.0 database is available at http://www.metabolicatlas.com in SBML (Systems Biology Mark-up Language) format. To construct a simulation-ready HMR 2.0 database, first it was tested so that all individual reactions, except pool reactions, were mass balanced. Second, it was guaranteed that high-energy compounds cannot be generated from low-energy compounds (such as ATP from ADP). This allowed us to test the thermodynamic constraints and the reversibility of the reactions. Third, the gap identification and gap-filling capabilities of the RAVEN Toolbox [23] were used to guide targeted literature studies to keep the number of dead-end reactions to a minimum. The production of all metabolites in the model was tested using artificial reactions ( Supplementary Data 10 ). Artificial reactions were used to ensure the connectivity and were not included during the simulations and network-dependent analysis. Consensus GEMs for hepatocytes GEMs provide biologically meaningful mechanistic basis for the genotype–phenotype relationships, yet it is necessary to have functional cell-type GEMs to identify the metabolic differences between different states. We reconstructed iHepatocytes2322 by merging recently generated GEM for hepatocytes iHepatocyte1154 and previously published liver models [1] , [15] , [21] , [22] . iHepatocyte1154 was generated from the HMR database using the INIT algorithm, which allows for automated reconstruction of GEMs based on the cell-type-specific proteome in the HPA ( http://www.proteinatlas.org ) [20] . We incorporated differentially expressed genes ( t -test, P -value <0.001) in NAFLD patients in our reconstruction process, as iHepatocytes2322 is used for the analysis of NAFLD patient data. Moreover, we integrated biochemical knowledge about hepatocyte metabolism and a large number of additional clinical data into the model. The resulting iHepatocytes2322 is the largest cell/tissue-type-specific GEM and contains 2,322 genes, 5,686 metabolites (2,895 unique metabolites) in 8 different compartments and 7,930 reactions. In the model, 74% of the reactions are associated to one or more genes. iHepatocytes2322 was validated with 256 known biological functions of hepatocytes ( Supplementary Data 5 ), based on the definitions by Gille et al . [1] , by using the checkTasks function in the RAVEN Toolbox [23] . Transcriptomics data for NAFLD To study the appearance of human NAFLD through the changes in global gene expression, microarray data for liver samples were retrieved from ArrayExpress public repository (accession code E-MEXP-3291 ). The data include samples from 45 different subjects and the samples were diagnosed as healthy ( n =19), steatotic ( n =10), NASH with FL ( n =9) and NASH without FL ( n =7) [34] . The age, gender and disease state of the patients are presented ( Supplementary Data 8 ). The steatotic samples did not demonstrate significant gene expression changes compared with normal samples, as similarly reported in the plasma metabolic profiling of subjects with NAFLD, steatosis and NASH [50] ( Supplementary Fig. 1 ). Hence, we performed the pair-wise comparison analysis of the gene expression to compare NASH with and without FL samples versus healthy ( Fig. 3 ) and steatotic ( Supplementary Fig. 2 ) samples using Piano R package [66] . Identified metabolic differences between the NAFLD patients through iHepatocytes2322 provided detailed information comparing the enrichment of differentially expressed genes in the KEGG pathways ( Supplementary Fig. 6 ). Differentially expressed genes in NASH with and without FL samples versus healthy and steatotic samples enriched in metabolism-related KEGG pathways, including steroid biosynthesis, oxidative phosphorylation, valine, leucine and isoleucine degradation, peroxisome, pyrimidine metabolism, pentose phosphate pathway and FA biosynthesis. Data availability HMR 2.0 database ( Supplementary Data 11 ) and GEM for hepatocytes iHepatocytes2322 ( Supplementary Data 12 ) is publically available in the SBML format at Human Metabolic Atlas ( http://www.metabolicatlas.org ). The annotation of the presence or absence of protein targets in hepatocytes together with the high-resolution images is publically available through the HPA ( http://www.proteinatlas.org ). How to cite this article: Mardinoglu, A. et al . Genome-scale metabolic modelling of hepatocytes reveals serine deficiency in patients with non-alcoholic fatty liver disease. Nat. Commun. 5:3083 doi: 10.1038/ncomms4083 (2014).